Structural basis for histone mimicry and hijacking of host proteins by influenza virus protein NS1 Pathogens can interfere with vital biological processes of their host by mimicking host proteins. The NS1 protein of the influenza A H3N2 subtype possesses a histone H3K4-like sequence at its carboxyl terminus and has been reported to use this mimic to hijack host proteins. However, this mimic lacks a free N-terminus that is essential for binding to many known H3K4 readers. Here we show that the double chromodomains of CHD1 adopt an ‘open pocket’ to interact with the free N-terminal amine of H3K4, and the open pocket permits the NS1 mimic to bind in a distinct conformation. We also explored the possibility that NS1 hijacks other cellular proteins and found that the NS1 mimic has access to only a subset of chromatin-associated factors, such as WDR5. Moreover, methylation of the NS1 mimic can not be reversed by the H3K4 demethylase LSD1. Overall, we thus conclude that the NS1 mimic is an imperfect histone mimic. Throughout evolution, histones are highly conserved proteins with a flexible N-terminal tail and the characteristic histone fold core domain. The N-terminal tails of histones, as well as more recently defined sites in the globular domain, can undergo post-translational modifications such as phosphorylation, acetylation and methylation. These modifications can be recognized by a large number of protein modules and consequently influence a multitude of cellular processes, including transcription, replication, DNA repair and cell cycle progression [1] . Pathogens often adapt to features of their hosts to gain functional advantage. A typical strategy is mimicry, in which pathogen proteins resemble host proteins to co-opt or disrupt host functions to the pathogen’s advantage [2] . Perfect mimics co-opt host functions to favour pathogen fitness, while imperfect mimics resemble host components but perform functions that are distinct from those of the host [2] . The non-structural protein 1 (NS1) of the influenza A H3N2 subtype, which is increasingly abundant in seasonal influenza and was the predominant subtype circulating in the past few seasons [3] , possesses a histone-like sequence that is used by the virus to target the human PAF1 transcription elongation complex [4] . The histone mimic in NS1 enables the influenza virus to selectively regulate inducible gene expression, thus contributing to suppression of the antiviral responses [4] . The NS1 protein of influenza A viruses is not a structural component of the virion, but is expressed at very high levels in infected cells [5] . It has multiple accessory functions during viral infection, including conferring resistance to antiviral interferon induction, replication, pathogenesis, virulence and host range adaption [5] . NS1 has two domains, an N-terminal RNA-binding domain and a C-terminal effector domain separated by a linker [6] . NS1 of the influenza A (H3N2) virus possesses the 226 ARSK 229 sequence at its carboxyl terminus that is analogous to the N-terminal 1 ARTK 4 sequence of histone H3 (referred to as 1 AR(T/S)K 4 motif thereafter) [4] . Notably, the C terminus of NS1 is non-structured and potentially highly interactive [6] , similar to the histone tail. The 1 ARTK 4 motif of H3 can undergo several post-translational modifications, including methylation at R2 and K4, and phosphorylation at T3 (ref. 1 ). These modifications can promote or impede binding of a large number of proteins [7] . The 226 ARSK 229 motif of NS1 can also be methylated and acetylated at lysine by host enzymes in vitro and in vivo [4] , mimicking histone H3 not only via sequence, but also via post-translational modifications. Indeed, CHD1 (chromodomain-helicase-DNA-binding protein 1), which binds H3K4me3 via its double chromodomains [8] , was identified as a methylation-dependent binder of NS1 (ref. 4 ). CHD1 is an ATP-dependent chromatin-remodeling factor and plays an important role in regulating nucleosome assembly and mobilization [9] . CHD1 possesses double chromodomains (CD1 and CD2) in its N-terminal region, a SWI2/SNF2 helicase/ATPase domain consisting of DEXDc and HELICc subdomains in the middle, and a DNA-binding domain consisting of SANT and SLIDE domains in its C-terminal region [10] . Human CHD1 was found to specifically recognize H3K4me3, a hallmark of actively transcribed chromatin, and to mediate subsequent recruitment of post-transcriptional initiation and pre-mRNA splicing factors [11] . Moreover, CHD1 has a critical role in the genome-scale replication-independent nucleosome assembly at the very early stage of development, as maternal CHD1 is required for the incorporation of histone H3.3 into the male pronucleus during decondensation after fertilization [12] . Many protein modules are able to bind methylated or unmethylated H3K4, including PHD fingers, Tudor domains and chromodomains [7] . Most of them require a free N terminus of histone H3 for recognition. However, the 226 ARSK 229 motif of NS1 is located at the C terminus of the protein, and therefore lacks the free N-terminal amine. We were interested in understanding how NS1 hijacks host proteins via this mimic. In the present study, by means of biophysical binding assays and X-ray crystal structure analysis, we reveal the molecular basis for NS1 mimicry of H3K4 and binding to CHD1. First, the double chromodomains of CHD1 adopt a shallow and open pocket to interact with the free N-terminal amine of H3K4, and this pocket could tolerate the NS1 mimic binding after a conformational change of the peptide. Second, CHD1 preferentially binds to the dimethylated 1 AR(T/S)K 4 motif. Third, the arginine residue within the 1 AR(T/S)K 4 motif plays a critical role in binding to CHD1, although its methylation status has limited effect. We also explored the possibility that NS1 hijacks other cellular proteins and identified a new potential target, WDR5, a common component of the coactivator complexes MLL, SET1A, SET1B, NLS1 and ATAC [13] . We conclude that due to its lack of a free N terminus, which is critical for histone H3K4 to recruit cellular effector proteins, NS1 could hijack only a specific subset of H3K4-binding proteins in its hosts. Furthermore, we found that methylation of NS1 mimic can not be reversed by the histone H3K4 demethylase LSD1, suggesting that it adopts a distinct regulation mechanism from that of histone H3K4me. Taken together, the NS1 mimic is an imperfect histone mimic. CHD1 preferentially recognizes dimethylated H3 and NS1 The double chromodomains of CHD1 have been reported to recognize methylated lysine 4 in the histone H3 N-terminal tail [8] . To determine the preference of CHD1 for different methylation states of H3K4, we performed isothermal titration calorimetry (ITC) assays using synthetic peptides and recombinant double chromodomain protein of CHD1. Our binding results display that the CHD1–H3K4 interaction is methylation dependent, and CHD1 preferentially recognizes the dimethylated H3K4 ( K d values: 14.5 μM (H3K4me3), 9.6 μM (H3K4me2), 21 μM (H3K4me1), 365 μM (H3K4me0) in a low salt buffer containing 20 mM Tris–HCl, pH 7.5, 50 mM NaCl, 1 mM DTT) ( Fig. 1a ). A similar trend was observed for the NS1 histone mimic ( K d values: 29 μM (NS1K229me3), 22 μM (NS1K229me2), >500 μM (NS1K229me0) in the same low salt buffer) ( Fig. 1b ). 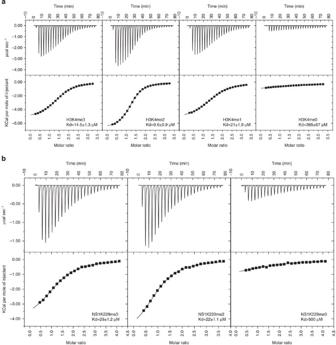Figure 1: CHD1 preferentially recognizes dimethylated H3 and NS1. ITC assays of CHD1 chromodomains with histone H3 peptides (a) and NS1 peptides (b) in a low salt buffer containing 20 mM Tris–HCl, pH 7.5, 50 mM NaCl, 1 mM DTT.Kdvalues were calculated from single measurement and errors were estimated by fitting curve. We also performed ITC in a higher salt concentration buffer (250 mM NaCl) and found that the high salt concentration slightly weakened the NS1/H3K4 peptide binding to CHD1 ( Table 1 and Supplementary Fig. 1 ). Taken together, our ITC assays indicate that the double chromodomains of CHD1 preferentially recognize the dimethylated AR(T/S)K motif, irrespective of the motif's N-terminal or C-terminal sequence context. Figure 1: CHD1 preferentially recognizes dimethylated H3 and NS1. ITC assays of CHD1 chromodomains with histone H3 peptides ( a ) and NS1 peptides ( b ) in a low salt buffer containing 20 mM Tris–HCl, pH 7.5, 50 mM NaCl, 1 mM DTT. K d values were calculated from single measurement and errors were estimated by fitting curve. Full size image Table 1 Full size table Structural basis for recognition of NS1 mimic by CHD1 A large number of histone readers have been found to recognize histone H3K4, and the free N-terminal amine of H3 plays a critical role in the specific recognition. For example, the PHD finger of ING4 (ref. 14 ) and the double Tudor domains of SGF29 (ref. 15 ) are two well established H3K4me3-binding modules. Acetylation of the N-terminal amine or addition of extra residues to the N terminus of the histone H3K4 peptide disrupts their binding to these histone-binding modules [14] , [15] . Consistently, neither ING4 nor SGF29 showed detectable binding to a corresponding NS1 peptide ( Table 1 ). Another example is Survivin, which specifically recognizes phosphorylated H3T3 and also requires the free N-terminal amine of H3 for interaction [16] . Why is CHD1 able to recognize the methylated 226 ARSK 229 motif of NS1 in a C-terminal context? 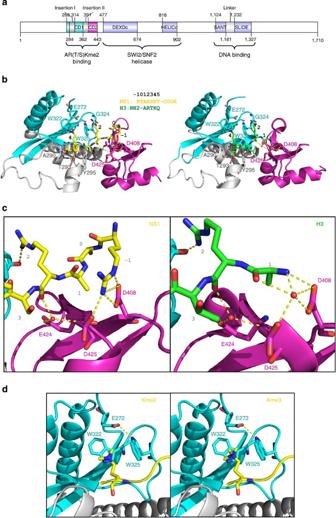Figure 2: Structural basis for the AR(T/S)K motif recognition by the double chromodomains of CHD1. (a) Domain organization of CHD1. (b) Overall structure of the double chromodomains of CHD1 in complex with a trimethylated NS1 peptide (left), and in complex with a trimethylated histone H3K4 peptide for comparison (right, PDB ID: 2B2W). (c) Detailed interactions of the residue A226(NS1)/A1(H3) with CHD1. (d) Comparison of Kme2 and Kme3 recognition by CHD1. To address this question, we solved the crystal structures of the double chromodomains of CHD1 bound to di- and tri-methylated NS1 peptides, respectively ( Table 2 and Supplementary Fig. 2a and b ). Table 2 Data collection and refinement statistics. Full size table The NS1 peptide binds to CHD1 mainly through two types of interactions ( Fig. 2 ). The first one is the cation-π interactions between the peptide’s methylated lysine and the two tryptophan residues, W322 and W325, from CHD1-CD1. These interactions are reinforced by E272 from CHD1-CD1 through formation of a negatively charged cage, interacting with the positively charged methyl-lysine. The second type of interactions involves a series of hydrogen bonding interactions, directly or mediated by an ordered solvent, between the peptide and CHD1. This is consistent with the ITC results showing that the binding affinity is dependent on the salt concentration. Although the NS1 peptide is located at the C terminus of the protein, the most C-terminal residue, V230, of the NS1 protein does not show any interactions with CHD1. Figure 2: Structural basis for the AR(T/S)K motif recognition by the double chromodomains of CHD1. ( a ) Domain organization of CHD1. ( b ) Overall structure of the double chromodomains of CHD1 in complex with a trimethylated NS1 peptide (left), and in complex with a trimethylated histone H3K4 peptide for comparison (right, PDB ID: 2B2W). ( c ) Detailed interactions of the residue A226(NS1)/A1(H3) with CHD1. ( d ) Comparison of Kme2 and Kme3 recognition by CHD1. Full size image Structural comparison reveals that the NS1–CHD1 complex structures are almost identical to the complex structure of CHD1 bound to a trimethylated histone H3 peptide, which has been reported previously [8] . The main structural differences arise between A226 of NS1 and A1 of H3, as well as the residues preceding A226 in NS1 ( Fig. 2c ). In the previously published histone H3 complex structure, the N-terminal amine of A1 is hydrogen bonded to D408 directly and to D425 via an ordered water molecule. In the NS1 complex structures, A226 (corresponding to A1 in H3) rotates about 60° to flip out the peptide and loses contact with the protein. Instead, the peptide adopts a turn so that the R224 (R-1) residue is able to form salt bridges with both D408 and D425 from CHD1-CD2. To further understand the structural basis for CHD1’s interactions with NS1, we compared these structures with those of ING4 and SGF29 bound to H3K4me3, and Survivin bound to H3T3ph. Notably, all of ING4, SGF29 and Survivin form a deep and negatively charged pocket to anchor the free N-terminal amine of H3, and any modification on the free N-terminal amine of H3A1 would disrupt binding ( Supplementary Fig. 3 ). In contrast, the H3A1 binding site of CHD1 is shallow and open, tolerating AR(T/S)K motif in different sequence contexts. Although NS1 has a similar ARSK motif as histone H3K4, the lack of a free N-terminal amine distinguishes it from histone H3. Consequently, not all H3K4-binding proteins can be hijacked by NS1. To rationalize preferential recognition of dimethylated lysine by CHD1, we superimposed and compared the complex structures of di- and tri-methylated NS1 peptides ( Fig. 2d ). In the case of the dimethylated lysine peptide, the two methyl groups of the dimethylated lysine face the CHD1 residue W322, leaving the hydrophilic –NH group exposed to solvent. For the trimethylated lysine, the third methyl group is unfavourably exposed to solvent. This selection mechanism differs from that of other dimethyl-lysine reader domains such as the Tudor domain of 53BP1 (ref. 17 ) and the MBT domains of L3MBTL1/2 (refs 18 , 19 ), in which an aspartic acid residue forms a salt bridge with the dimethyl-lysine ammonium group, totally excluding a third methyl group. R2 plays a critical role in CHD1 binding to the ARTK motif To evaluate the relative importance of each residue in the 1 ARTK 4 motif to bind CHD1, we designed a peptide array in which residues around K4me2 were substituted with each of the 20 amino acids. This array was then probed for CHD1 binding ( Fig. 3a ). First, negatively charged residues (Asp and Glu) were not allowed at any positions examined. This was expected, as the peptide binding surface of CHD1 is largely negatively charged ( Fig. 3b ). Second, substitution of R2 by any other residue except lysine abolished binding to CHD1, whereas substitutions at other positions had limited effect on binding. Consistently, the R2A mutant peptide of histone H3K4me2 exhibited a dissociation constant of ~\n164 μM in 50 mM NaCl buffer, which was 16-fold weaker than the H3K4me2 peptide ( Fig. 3c ). This indicates that R2 plays a critical role in the 1 AR(T/S)K 4 motif for protein binding. 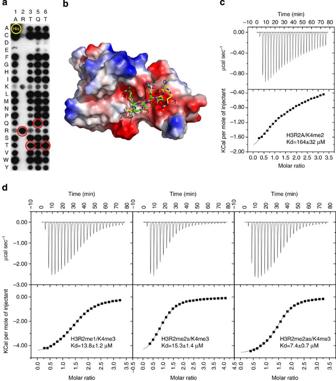Figure 3: The R2 residue of the histone H3K4 peptide plays a critical role in binding to the double chromodomains of CHD1. (a) Peptide array for CHD1 binding. Peptide sequences are based on the H3K4me2 sequence: ART(Kme2)QT. In each column the corresponding wild-type residue was substituted with each of the 20 amino acids. The AA position is an 8 × His peptide, served as a positive control. Red circles represent wild-type sequences. (b) Electrostatic potential (isocontour value of ±76kT/e) surface representation of the CHD1 bound to the trimethylated NS1 (yellow) or H3K4 (green) peptides. (c,d) ITC results for CHD1 with indicated peptides in a low salt buffer containing 20 mM Tris–HCl, pH 7.5, 50 mM NaCl, 1 mM DTT.Kdvalues were calculated from single measurement and errors were estimated by fitting curve. Figure 3: The R2 residue of the histone H3K4 peptide plays a critical role in binding to the double chromodomains of CHD1. ( a ) Peptide array for CHD1 binding. Peptide sequences are based on the H3K4me2 sequence: ART(Kme2)QT. In each column the corresponding wild-type residue was substituted with each of the 20 amino acids. The AA position is an 8 × His peptide, served as a positive control. Red circles represent wild-type sequences. ( b ) Electrostatic potential (isocontour value of ±76 kT / e ) surface representation of the CHD1 bound to the trimethylated NS1 (yellow) or H3K4 (green) peptides. ( c , d ) ITC results for CHD1 with indicated peptides in a low salt buffer containing 20 mM Tris–HCl, pH 7.5, 50 mM NaCl, 1 mM DTT. K d values were calculated from single measurement and errors were estimated by fitting curve. Full size image Arginine can be mono-, asymmetric or symmetric di-methylated in vivo , and these modifications can have different effects on protein binding and consequently on biological function [21] . We performed a series of ITC assays using peptides of different R2 methylation states in a trimethylated K4 context and found that R2 methylation status had limited effect on binding to CHD1 ( Fig. 3d , Table 1 ). Methylation of NS1 can not be reversed by LSD1 Methylation of histone H3K4 is dynamically regulated by lysine methyltransferases and demethylases [1] . The NS1 histone mimic can be methylated by methyltransferase Set1 complex and Set7/9 (ref. 4 ). However, it was unclear whether the resultant methylation can be reversed or not. Methylated histones can be demethylated by two families of enzymes, amine oxidases such as LSD1 and the JmjC family of hydroxylases [1] . Structural studies reveal that a free N terminus of H3 is required for the H3K4me2 demethylation by LSD1/2 (refs 22 , 23 ), suggesting that the NS1 mimic could probably escape from the regulation of these demethylases. To confirm this, we carried out demethylase assays. Namely, we incubated the dimethylated NS1 peptide with purified active LSD1 demthylase, and the reaction mixtures were analysed by mass spectrometry. As controls, the H3K4me2 and H3K4me1 peptides were completely converted to the unmethylated product: H3K4me0 on incubation with LSD1 ( Fig. 4a ). In contrast, the dimethylated NS1 peptide was found to be not demethylated by LSD1 ( Fig. 4b ), indicating that methylation of NS1 can not be reversed by LSD1. 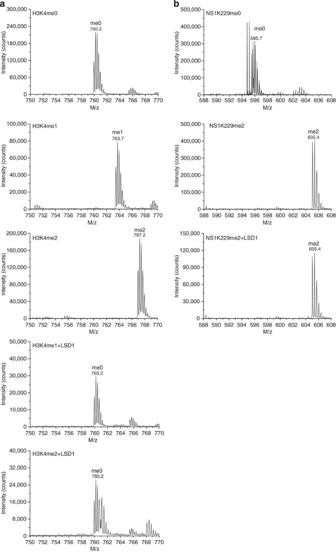Figure 4: Metylation of NS1 can not be reversed by LSD1. Mass spectrometry results of H3K4 (a) or NS1 (b) peptides after incubation with buffer or purified LSD1 protein. Them/zsignals for the +4-charged peptides are shown. Figure 4: Metylation of NS1 can not be reversed by LSD1. Mass spectrometry results of H3K4 ( a ) or NS1 ( b ) peptides after incubation with buffer or purified LSD1 protein. The m/z signals for the +4-charged peptides are shown. Full size image ARTK motif binding ability of the CHD family chromodomains The CHD family includes nine members, CHD1~\n9, and each of them contains tandem double chromodomains. However, with the exception of CHD1 (refs 8 , 11 ), the functional role of CHD chromodomains remains unclear. Here we combined sequence and structure analysis with fluorescence polarization binding assays to explore their histone-binding ability. Sequence alignment revealed that these chromodomains can be divided into three subfamilies: CHD1/2, CHD3/4/5 and CHD6/7/8/9 ( Fig. 5a ) [24] . Although CHD2 exhibits high sequence identity to CHD1, we did not observe any binding between CHD2 and the methylated histone H3K4 peptides using FP ( Fig. 5b ). 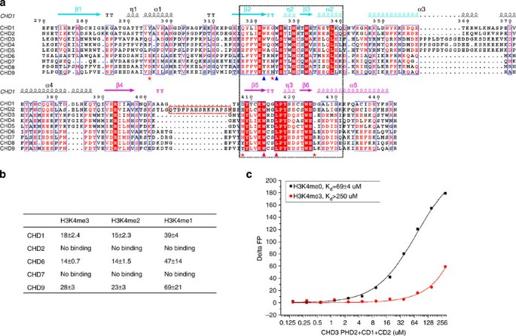Figure 5: Histone-binding ability of the double chromodomains from CHD family. (a) Sequence alignment of the double chromodomains for all human CHD members. Secondary structural elements of CHD1 are shown above the sequences. Cyan, CD1; Magenta, CD2. Blue triangles, aromatic residues involved in methyl-lysine recognition in CD1; red triangles, corresponding residues in CD2 to the blue triangle residues in CD1; red star, other key residues for CHD1 binding to the AR(T/S)K motif. (b) Dissociation constants (μM) of the double chromodomains of some CHD proteins to different H3K4 peptides measured by FP. (c) FP binding curves for the PHD2-double chromodomains of CHD3. (b,c)Kdvalues were calculated from single measurement and errors were estimated by fitting curve. Figure 5: Histone-binding ability of the double chromodomains from CHD family. ( a ) Sequence alignment of the double chromodomains for all human CHD members. Secondary structural elements of CHD1 are shown above the sequences. Cyan, CD1; Magenta, CD2. Blue triangles, aromatic residues involved in methyl-lysine recognition in CD1; red triangles, corresponding residues in CD2 to the blue triangle residues in CD1; red star, other key residues for CHD1 binding to the AR(T/S)K motif. ( b ) Dissociation constants (μM) of the double chromodomains of some CHD proteins to different H3K4 peptides measured by FP. ( c ) FP binding curves for the PHD2-double chromodomains of CHD3. ( b , c ) K d values were calculated from single measurement and errors were estimated by fitting curve. Full size image The CHD3/4/5 subfamily loses an aromatic residue for methyl-lysine binding at the position corresponding to W325 of CHD1 ( Fig. 5a ), suggesting that they may lose the ability to bind methylated histones. In contrast, there are two tandem PHD fingers preceding the double chromodomains in CHD3/4/5, which can interact with unmethylated histone H3K4 (refs 25 , 26 ). Because the construct covering the double chromodomains of CHD3 was insoluble, we used a construct covering PHD2 and the double chromodomains for FP assays. This construct was able to bind to the unmodified peptide H3K4me0 with a K d of ~\n69 μM as expected from its PHD domain, but showed just marginal binding to the H3K4me3 peptide ( Fig. 5c ), confirming that the double chromodomains in the CHD3/4/5 subfamily lose the ability to bind H3K4me2/3. The CHD6/7/8/9 subfamily harbours tyrosine or phenylalanine at the positions corresponding to the aromatic cage (W322 and W325) of CHD1, suggesting that potentially they might bind methyl-lysine. The constructs of the double chromodomains of CHD6/7/9 were soluble and were consequently used for binding assays. Indeed, CHD6/9 showed modest binding affinity to H3K4me3/2, whereas no interaction was observed for CHD7 ( Fig. 5b ). We then examined the binding ability of CHD6/9 towards the NS1 mimic using ITC assays. However, neither showed detectable interactions ( Table 1 ), suggesting that imperfection of NS1 mimic prevents it from hijacking these CHD proteins. WDR5 is a new potential target of NS1 R2 of histone H3 serves as a key binding site for WDR5 (refs 27 , 28 ), a common component of the coactivator complexes MLL, SET1A, SET1B, NLS1 and ATAC. Given the critical role of R2 in the 1 AR(T/S)K 4 motif, we were interested in whether the NS1 mimic could bind to WDR5. Our ITC assay indeed showed a modest interaction between WDR5 and the unmodified NS1 peptide with a dissociation constant of ~\n70 μM ( Fig. 6a ). We also succeeded in crystallizing the complex of WDR5 bound to the NS1 peptide and solving the complex structure ( Fig. 6b , Table 2 and Supplementary Fig. 2c ). The electron density for an arginine residue and the surrounding peptide backbone was clearly observed. Poor side chain density for surrounding residues prevented conclusive assignment of the residue number of the arginine residue, as there were three arginine residues in the peptide ( Fig. 6c ). A binding mode where WDR5 is not bound to the 226 ARSK 229 motif of NS1 but switches to the preceding 223 ARTA 226 motif ( Fig. 6c ) is therefore possible. Nevertheless, it is safe to say that the NS1 peptide binding by WDR5 is mainly attributed to an arginine residue in the peptide ( Supplementary Fig. 2c ), similar to previous findings from the WDR5-H3 structures [27] , [28] ( Fig. 6b,d ). The peptide binding cleft of WDR5 is very plastic and can bind to a variety of arginine containing peptides, including its own arginine containing N-terminal tail, epitope His-tag fused to WDR5 and Win motifs from the SET1 family [27] , [29] . Hence, the arginine is the major structural determinant for WDR5 binding. 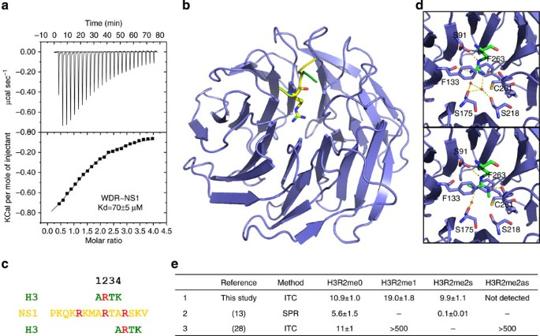Figure 6: The NS1 AR(T/S) motif is recognized by WDR5. (a) ITC binding curves of WDR5 and the unmodified NS1 peptide. (b) Overall structure of WDR5 in complex with the NS1 peptide (yellow), compared with the histone H3 peptide (green, PDB ID: 2H13). (c) Two AR(T/S) motifs are present in the NS1 C terminus. (d) Comparison of the Rme0 (top, PDB ID: 2H13) and Rme2s (down, PDB ID: 4A7J) peptides recognition by WDR5. (e) Dissociation constants (μM) of WDR5 to histone H3R2 peptides with different methylation states. (a,e)Kdvalues were calculated from single measurement and errors were estimated by fitting curve. Figure 6: The NS1 AR(T/S) motif is recognized by WDR5. ( a ) ITC binding curves of WDR5 and the unmodified NS1 peptide. ( b ) Overall structure of WDR5 in complex with the NS1 peptide (yellow), compared with the histone H3 peptide (green, PDB ID: 2H13). ( c ) Two AR(T/S) motifs are present in the NS1 C terminus. ( d ) Comparison of the Rme0 (top, PDB ID: 2H13) and Rme2s (down, PDB ID: 4A7J) peptides recognition by WDR5. ( e ) Dissociation constants (μM) of WDR5 to histone H3R2 peptides with different methylation states. ( a , e ) K d values were calculated from single measurement and errors were estimated by fitting curve. Full size image Methylation status on H3R2 affects binding to WDR5 (refs 13 , 28 , 30 ), but this relationship has never been systematically and quantitatively assessed. Here, we used the ITC binding assay to determine the binding affinities of WDR5 to peptides carrying different H3R2 methylation states. We found that mono- and symmetric di-methylation had limited effect on the binding affinity (19 μM and 9.9 μM versus 10.9 μM for unmethylated arginine), whereas asymmetric dimethylation abolished the interaction ( Fig. 6e and Supplementary Fig. 4 ). Structurally, the symmetric dimethylated arginine would introduce hydrophobic interactions with F133 and F263 of WDR5 via its methyl groups, but, at the same time, it would also lose two hydrogen bonds to the protein, compared with the unmethylated arginine ( Fig. 6d ) [13] . It has been well established that pathogen mimics interfere with important cellular processes, including cell growth and survival, cytoskeletal dynamics, membrane traffic and immune-related functions [2] . Recently, an NS1 histone mimic was reported to be able to hijack the human PAF1 transcription elongation complex and control antiviral gene expression [4] . In the present study, we have uncovered the structural basis for influenza virus NS1 mimicry of histone H3K4 and the hijacking of host proteins CHD1 and WDR5. CHD1 is a chromatin-remodelling factor and can mediate recruitment of post-transcriptional initiation and pre-mRNA splicing factors [11] . Importantly, in pancreatic cancer cells, expression and nuclear transport of CHD1 are regulated by the core subunit of PAF1 complex [31] , and there is also direct interaction between CHD1 and PAF1 (ref. 31 ), revealing cooperation between the CHD1 and transcription elongation. WDR5 is a core subunit of the human MLL and SET1 histone H3K4 methyltransferase complexes and is required for global H3K4 methylation as well as HOX gene activation in human cells [32] . Both CHD1 and WDR5 have critical role in regulation of gene expression. NS1 also can affect host gene expression by interfering with RNA splicing and messenger RNA export [33] , [34] . By mimicking histone H3, the H3N2 influenza A virus gains access to histone-interacting transcriptional regulators that control inducible antiviral gene expression. However, further study is needed to investigate the detailed mechanism by which NS1 suppresses antiviral responses through hijacking of CHD1 and WDR5. The 1 ARTK 4 motif of H3 locates at the N terminus of the protein. So far, dozens of protein modules have been identified as readers of this motif and its modification, including Tudor domain, Chromodomain, WD40 domain, PHD finger and CW domain [7] . Most of them recognize not only the sequence but also the free N-terminal amine of the motif. Any modification of the N-terminal amine or addition of extra residues to the N terminus of the histone H3K4 peptide would impede partners from binding. The NS1 histone mimic is located at the C terminus of the protein, therefore lacking a free amine. This feature confers it as an imperfect mimic. Subsequently, NS1 can hijack only a subset of H3K4-binding proteins of host and perform functions in a more selective manner. Our binding assays performed with peptides reveal that the NS1 mimic has slightly weaker binding to CHD1 than the histone H3K4 peptides, although we cannot exclude the possibility that the full-length NS1 has stronger binding affinity to CHD1. Interestingly, similar to the N-terminal histone H3 tail, the NS1 C terminus is also predicted to be unstructured. Furthermore, while host factors commonly fall under the regulation of cellular processes that control their activity, pathogens often can escape from cellular regulation by imperfect mimicry. Indeed, while methylation of H3K4 is under dynamic regulation by both methyltransferases and demethylases [1] , methylation of NS1 histone mimic can not be reversed by histone H3K4 demethylase LSD1, at least partially escaping from the host regulation. In conclusion, imperfect mimicry is generally more advantageous to pathogens, because effective mimics do not just mirror host functions but also subvert cellular processes to favour pathogen fitness [2] . Protein expression and purification The following constructs were cloned into the pET28a-MHL vector: CHD1 (aa 268–443), CHD2 (aa 260–452), CHD3 (aa 499–759), CHD6 (aa 285–435), CHD7 (aa 790–950), CHD9 (aa 680–840), ING4 (aa 184–248), SGF29 (aa 115–293) and WDR5 (aa 24–334). Recombinant proteins were expressed in an SGC-generated derivative strain of BL21 Escherichia coli with the pRARE plasmid for overcoming the codon bias. Cells were grown in TB media in the presence of kanamycin and chloramphenicol at 37 °C to an optical density of ~\n2. Protein expression was induced with 0.5 mM isopropyl-1-thio-β- D -galactopuranoside (IPTG) at 16 °C, and the cell cultures were harvested ~\n16 h after induction. Proteins were purified by a Ni-NTA column (Qiagen) followed by a gel filtration column (Superdex 75, GE Healthcare). For WDR5, His-tag was removed by using the TEV protease. Isothermal titration calorimetry The proteins were diluted into 20 mM Tris–HCl buffer (pH 7.5) containing 50 mM or 250 mM NaCl and 1 mM DTT. Lyophilized H3 peptides were dissolved in 20 mM Tris–HCl buffer containing 150 mM NaCl to a concentration of around 100 mM, and the pH was adjusted to 7.5 by adding NaOH. ITC measurements were carried out with protein and ligand concentrations ranging from 50 to 100 μM and 1–2 mM, respectively, in a VP-ITC instrument at 20 °C. Binding constants were calculated by fitting the data using the ITC data analysis module of Origin 7.0 (OriginLab Corp.). Fluorescence polarization assay All peptides used for fluorescence polarization measurements were synthesized C terminally labelled with fluorescein isothyocyanate and purified by Tufts University Core Services. Binding assays were performed at 20 °C in 20 μl volume at a constant labelled peptide concentration of 40 nM and with increasing amounts of proteins at concentrations ranging from low to high micromolar in 20 mM Tris pH 7.5, 150 mM NaCl, 1 mM DTT. Fluorescence polarization assays were performed in 384-well plates, using the Synergy 2 microplate reader (BioTek). An excitation wavelength of 485 nm and an emission wavelength of 528 nm were used. The data were corrected for background of the free labelled peptides. To determine K d values, the data were fit to a hyperbolic function using OriginPro 7.5 software (OriginLab Corp.). Peptide array binding assay Peptides were synthesized directly on a modified cellulose membrane with a polyethylglycol linker using the peptide synthesizer MultiPep (Intavis). The degenerate peptide library consisted of 100 membrane-immobilized peptides corresponding to control peptides and 6-residue-long stretches of histone H3 sequences corresponding to residues 1–6. The lysine at positions 4 was always dimethylated, whereas flanking residues were systematically substituted with each of the 20 L -amino acids. The binding assay was performed as described previously [35] . In brief, the membrane was extensively blocked with skim milk, incubated overnight with 5 μM 6 × His-tagged double chromodomains of CHD1, washed with PBS/Tween and visualized via western blot analysis with an anti-His antibody (Abcam, ab184607, 2000 × dilution). Demethylation assay Mass spectrometry analysis was performed to determine whether LSD1 was capable of demethylating dimethylated NS1 (NS1K229me2). The reactions (40 μl final volume) contained 0.5 mM of each corresponding peptide and 1 μM LSD1 (Cat #:50097; BPS bioscience) in buffer containing 20 mM Tris–HCl, pH 8.0 and 0.01% Triton X-100. The reactions were incubated overnight at 37 °C, quenched by addition of 110 μl of 0.5% formic acid and immediately frozen on dry ice. A reaction mixture with no LSD1 was used as a control for every experiment. The samples were analysed by an Agilent LC/MSD Time-Of-Flight (TOF) mass spectrometer (Agilent Technologies, Santa Clara, CA, USA) equipped with an electrospray ion source. To separate the peptide from the protein and remove buffer and salt, the samples were passed through a POROSHELL 300SB-C3 column using a 5–95% acetonitrile:water gradient. Protein crystallization Purified proteins mixed with a three- to fivefold stoichiometric excess of the respective peptides were crystallized using the sitting drop vapor diffusion method at 18 °C by mixing 0.5 μl of the protein with 0.5 μl of the reservoir solution. The CHD1-NS1K229me2 complex was crystallized in 15% PEG3350, 0.1 M succinate, pH 7.0; the CHD1-NS1K229me3 complex was crystallized in 10% PEG 8000, 0.2 M MgCl 2 , 0.1 M Tris buffer at pH 8.5; the WDR5-NS1(unmodified) complex was crystallized in 25% PEG3350, 0.1 M (NH 4 ) 2 SO 4 , 0.1 M Bis-Tris pH 6.5. Data collection and structure determination All crystals were transferred to a reservoir solution with 15% (v/v) glycerol as cryoprotectant before flash freezing in liquid nitrogen. For WDR5-NS1 and CHD1-NS1K229me3 crystals, data collection was performed at beamline 19ID of the APS synchrotron at 0.9792 Å and 0.9793 Å, respectively. For the CHD1-NS1K229me2 crystal, data collection was performed at a Rigaku FR-E system at 1.5418 Å. All data sets were collected at 100 K. All diffraction patterns were indexed, integrated with XDS [36] and scaled with AIMLESS [37] . The structures were solved by molecular replacement with PHASER [38] . An unpublished WDR5 model was used to solve the WDR5 complex structure, and coordinates derived from PDB entry 2B2W [8] were used to solve the CHD1 complexes. Coot [39] was used for interactive model building. Molprobity [40] was used for model geometry validation. Final model refinement was performed with PHENIX [41] for the CHD1-NS1K229me3 complex and REFMAC [42] for the other two complexes. Compilation of data and crystallographic models for statistical summary and PDB deposition were aided by PDB_EXTRACT [43] and IOTBX [44] . Ramachandran statistics were as follows: CHD1-NS1K229me3 complex structure, 95.0% in favoured regions, 5.0% in additional allowed regions, 0% generously allowed regions; CHD1-NS1K229me2 complex structure, 95.4% in favoured regions, 4.6% in additional allowed regions, 0% generously allowed regions; WDR5-NS1 complex structure, 87.4% in favoured regions, 12.2% in additional allowed regions, 0.4% generously allowed regions. No residues were in disallowed regions for all these structures. Accession code: Coordinates and structural factors are deposited in the Protein Data Bank under the following accession numbers: double chromodomains of CHD1 in the NS1-bound states: 4NW2 and 4O42 ; WDR5 in the NS1-bound state: 4O45 . How to cite this article: Qin, S. et al. Structural basis for histone mimicry and hijacking of host proteins by influenza virus protein NS1. Nat. Commun. 5:3952 doi: 10.1038/ncomms4952 (2014).